Palladium-catalyzed regiodivergent hydrochlorocarbonylation of alkenes for formation of acid chlorides Novel strategy for acid chlorides formation that do not use carboxylic acids is particularly attractive in chemical synthesis but remains challenging. Herein, we reported the development of a highly effective Pd-catalyzed hydrochlorocarbonylation of alkenes with CO for the formation of alkyl acid chlorides. Chlorosilane and AcOH were found as a mild HCl source for the reaction. The reaction shows broad substrate scope and produces both branched and linear alkyl acid chlorides in good to high yields upon different ligands and solvents. Cooperating with follow-up acylation reactions, the Pd-catalyzed hydrochlorocarbonylation offers a complementary platform for the synthesis of diverse carbonyl compounds from alkenes. Mechanistic investigations suggested that the reaction proceeded though a palladium hydride pathway, and CO prompted reductive elimination of the acyl-Pd-Cl intermediate. The acid chlorides are one of the most versatile and useful building blocks, which have been widely applied in esters or amides formation, Friedel-Craft acylation, cross-couplings, polymerizations and many so forth [1] . Conventionally, they are synthesized through chlorination of carboxylic acids with SOCl 2 , PCl 3 , POCl 3 , (CO) 2 Cl 2 or other chlorinating reagents (Fig. 1a ) [2] , [3] . Nevertheless, heavily dependent on carboxylic acids as the substrates often limits the availability of the desired acid chlorides in target-oriented synthesis, that is especially true in the case of carboxylic acids were inaccessible. As a result, the direct conversion of organic functional groups into the synthetically useful acid chlorides is of great significance in chemical synthesis [4] , [5] . Recently, palladium-catalyzed chlorocarbonylations of aryl halides using CO as a cheap and readily available C1 source for the formation of aryl acid chlorides have been developed by Arndtsen and coworkers [6] , [7] , [8] , [9] . Palladium-catalyzed isodesmic shuttle reaction of unsaturated hydrocarbons and butyryl chloride to afford acid chlorides has been developed by Morandi and coworkers [10] , [11] , [12] . Notwithstanding, the development of novel and general strategies to access various alkyl acid chlorides from readily available starting materials remain highly desirable. Fig. 1: New strategies for acid chlorides’ formation. a Traditional methods for the synthesis of acid chlorides. b The original Pd-catalyzed hydrochlorocarbonylation of alkenes (1975). c Our work: Pd-catalyzed regiodivergent hydrochlorocarbonylation of alkenes with chlorosilane and AcOH. R, alkyl or aryl. Full size image Palladium-catalyzed hydrocarbonylations of alkenes represent a fundamental and powerful tool for the formation of carbonyl compounds [13] , [14] , [15] . With different nucleophiles in the reaction, the hydrocarbonylations create diverse carbonyl compounds such as amides [16] , [17] , [18] , [19] , [20] , [21] , [22] , [23] , esters [24] , [25] , [26] , [27] , [28] , [29] , [30] , [31] , [32] , and carboxylic acids [33] , [34] , [35] , [36] , [37] , [38] , [39] , [40] , with full atom economy. In this context, hydrochlorocarbonylation, a palladium-catalyzed hydrocarbonylation of alkenes with CO and HCl is supposed to be a possible approach to access acid chlorides in theory. However, distinct from the aminolysis/alcoholysis/hydrolysis of the key acyl-Pd-X intermediates in traditional hydrocarbonylations, the chlorolysis of the acyl-Pd-X species is considered be less likely due to the weak nucleophilicity of HCl. Whereas reductive elimination of the acyl-Pd-Cl species is assumed to form acid chlorides, the generated high reactive acid chlorides are readily undergo re-oxidative addition to palladium(0) catalyst [41] , [42] , thus leading to the hydrochlorocarbonylation proceeded in very low efficiency and with uncontrollable regioselectivity (Fig. 1b ) [43] , [44] . Moreover, the inevitable side hydrochlorination of alkenes by HCl (even became predominant reaction) is also importantly burned off the yield of desired acid chloride [43] , [44] . As a result, the original hydrochlorocarbonylation reaction has less been used in organic synthesis and less been known in the past half-century. Aiming to gain new and flexible methods for the formation of synthetically important alkyl acid chlorides, and based on our interest on palladium-catalyzed hydrocarbonylations [16] , [17] , [18] , [33] , herein, we report the development of a highly effective palladium-catalyzed regiodivergent hydrochlorocarbonylation of alkenes with CO (Fig. 1c ). 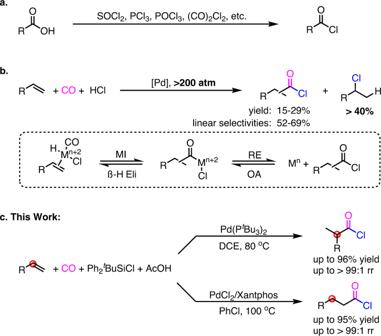Fig. 1: New strategies for acid chlorides’ formation. aTraditional methods for the synthesis of acid chlorides.bThe original Pd-catalyzed hydrochlorocarbonylation of alkenes (1975).cOur work: Pd-catalyzed regiodivergent hydrochlorocarbonylation of alkenes with chlorosilane and AcOH. R, alkyl or aryl. Optimization of reaction conditions We initiated the investigations of Pd-catalyzed hydrochlorocarbonylation with styrene 1a as the substrate at 80 °C in DCE under CO (Table 1 ). With Pd(PPh 3 ) 2 Cl 2 as the catalyst, the mixture of regioisomers of acid chlorides 2a/3a were indeed observed in 15% yield in the presence of HCl (entry 1). Unfortunately, due to the unavoidable hydrochlorination side-reaction initiated by HCl, the yield and regioselectivity of the reaction could not be improved after several attempts. We hypothesized that using in situ generated HCl might partially overcome the undesired hydrochlorination side reaction [45] . Therefore, a number of protocols for in situ formation of HCl have been examined in the reaction (entries 2–5) [46] . A 22% yield of acid chlorides 2a/3a were obtained with Ph 2 t BuSiCl/EtOH as the HCl source (entry 5). Nevertheless, the drawback of this Ph 2 t BuSiCl/EtOH reagent is of the accompanied hydroethanoxycarbonylation side reaction caused by EtOH. To this end, the Ph 2 t BuSiCl/AcOH reagent was found to be the best choice for hydrochlorocarbonylation, afford acid chlorides 2a/3a in 39% yields (entry 6). Table 1 Optimization of the reaction conditions a Full size table Since reductive elimination of the acyl-Pd(L)-Cl species might be a key factor of the reaction efficiency, various ligands, which might improve the reactivity and tune the regioselectivity of the reaction, were screened (entries 7–15). We were found that the use of monophosphines favors to access branched acid chloride 2a , while the use of bisphosphine ligands favors to access linear product 3a [47] . In this context, the sterically bulky P t Bu 3 showed the highest efficiency for the formation of the branched acid chloride 2a , thus offering the optimal conditions for branched selective hydrochlorocarbonylation of alkenes (entry 11). In contrast, although the linear acid chloride 3a was observed as the main product in the presence of Xantphos ligand, the yield and regioselectivity remains to be improved at this stage (entry 14). Therefore, other parameters including solvents, temperatures and pressure of CO were extensively optimized. After many attempts, a 95% yield of acid chloride 3a with l/b = 95:5 was finally obtained by using chlorobenzene as the solvent at 100 °C (entry 19). Hydrochlorocarbonylation of alkenes With the optimized reaction conditions in hand, the scope of the hydrochlorocarbonylation have been explored (Fig. 2 ). Under the conditions for the synthesis of branched acid chlorides, Pd-catalyzed hydrochlorocarbonylation of aryl alkenes proceeded well to give rise to the corresponding products in high yields with excellent regioselectivities (Fig. 2a ). The functional group tolerance of the reaction is of broad. Both electron-donating and electron-withdrawing groups, such as alkyl, alkoxyl, [1,3]-dioxol, F-, Cl-, Br-, CF 3 -, MeO 2 C-, sulfonyl, and even coordinative cyano-, were compatible under the conditions ( 2b-2o ). In addition, 2-vinylthiophene and vinylnaphthalenes were tolerated in the reaction to afford the desired acid chlorides 2p–2r in good to high yields. In contrast, under the conditions for the synthesis of linear acid chlorides, Pd-catalyzed hydrochlorocarbonylation of aryl alkenes also proceeded well to generate the corresponding linear acid chlorides in high yields with high regioselectivities (Fig. 2b ). The substrate scope and functional group tolerance in these cases ( 3b–3r ) were as good as the branched selective hydrochlorocarbonylation. Fig. 2: Pd-catalyzed regiodivergent hydrochlorocarbonylation of aryl alkenes. a Conditions: alkene (0.2 mmol), Pd(P t Bu 3 ) 2 (5 mol%), Ph 2 t BuSiCl (0.3 mmol), AcOH (0.3 mmol), CO (30 atm), DCE (1.5 mL), 80 °C, 24 h. b Conditions: alkene (0.2 mmol), PdCl 2 (5 mol%), Xantphos (6 mol%), Ph 2 t BuSiCl (0.3 mmol), AcOH (0.3 mmol), CO (40 atm), PhCl (1.5 mL), 100 °C, 24 h. c 100 °C. Yields refer to isolated yields of the derivatized methyl carboxylates (see SI). The ratios of regioisomers within parentheses were determined by GC-MS analysis of their derivatized methyl carboxylates of crude acid chlorides. Full size image The substrate scope with respect to alkyl alkenes was investigated (Fig. 3 ). The linear selective hydrochlorocarbonylation of alkyl alkenes were proceeded well, while the branched selective reaction was unsuccessful under the above standard conditions. As such, both non-functionalized alkenes and functionalized alkenes including lilestralis-derived alkene, 6-chlorohex-1-ene, 6-bromohex-1-ene, pent-4-enoic acid were proceeded under the linear selective conditions to form the carbon chain extended acid chlorides 4a–4h in high yields. With a bulky substituent adjacent to the alkene group, the regiomeric ratios (l:b) of products 4c–4e could be as high as >99:1. Expectedly, with 1,1-dialkyl substituted alkenes, 1-aryl-1-alkyl substituted alkenes, or exocyclic alkenes as the substrate, the corresponding acid chlorides 4i–4p were obtained in 70–86% yields. Fig. 3: Pd-catalyzed hydrochlorocarbonylation of various alkenes. Conditions: alkene (0.2 mmol), PdCl 2 (5 mol%), Xantphos (6 mol%), Ph 2 t BuSiCl (0.3 mmol), AcOH (0.3 mmol), CO (40 atm), PhCl (1.5 mL), 100 °C, 24 h. Isolated yields of the derivatized products (see SI). The ratio of isomers within parentheses was determined by GC-MS analysis of the derivatized products of the acid chlorides. Full size image Cyclic internal alkenes were feasible substrates in the reaction to form the desired acid chlorides 4q–4y in good to high yields. Whereas the isomerization of the alkyl substituted alkenes is typical a low energy barrier pathway in traditional hydrofunctionalizations [48] , [49] , [50] , the desired acid chlorides 4r–4v were obtained as the sole products in high yields. These results indicated that the insertion of [PdH] species into the double bond of the alkenes is irreversible in our hydrochlorocarbonylation. Notably, acenaphthylene and androstenone were tolerated in the reaction to afford the corresponding acid chloride 4x–4y in 65% to 71% yield. Synthetic application of hydrochlorocarbonylation The efficiency of above Pd-catalyzed hydrochlorocarbonylation encouraged us to establish a complementary platform for the synthesis of diverse carbonyl compounds from alkenes in one-pot manner (Fig. 4 ). In this respect, although the transformation of alkenes to esters and amides have been developed as exemplified by Pd-catalyzed hydroalkoxycarbonylation and hydroaminocarbonylation, the substrate scope of these reactions is often limited in primary alcohols and anilines [13] , [14] , [15] , [16] , [17] , [18] , [19] , [20] , [21] , [22] , [23] , [24] , [25] , [26] , [27] , [28] , [29] , [30] , [31] , [32] , [33] , [34] , [35] , [36] , [37] , [38] , [39] , [40] . Tertiary alcohols, phenols and aliphatic amines are typically incompatible with the traditional hydrocarbonylations because of their steric encumbrance, weak nucleophilicity, and strong basicity. Therefore, one-pot hydrochlorocarbonylation of alkenes and esterification with sterically encumbered alcohols or weakly nucleophilic phenols for the synthesis of corresponding esters has been explored. As illustrated in Fig. 4a , sterically encumbered bioactive alcohols, such as (-)-isopulegol, 19-hydroxyandrostendione, and lanosterol, were well tolerated in one-pot reactions to afford the desired esters 5a–5c and 6a–6c in good to high yields. Tertiary butanol and weakly nucleophilic phenol and estrone were also tolerated in one-pot reactions to form the corresponding esters 5d–5f and 6d–6f in good yields. 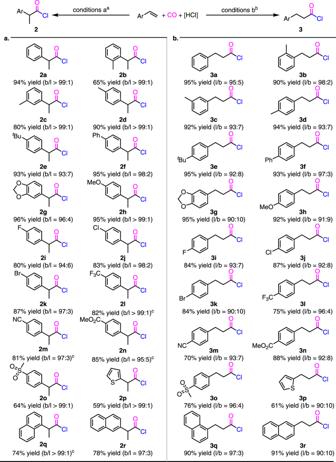Fig. 2: Pd-catalyzed regiodivergent hydrochlorocarbonylation of aryl alkenes. aConditions: alkene (0.2 mmol), Pd(PtBu3)2(5 mol%), Ph2tBuSiCl (0.3 mmol), AcOH (0.3 mmol), CO (30 atm), DCE (1.5 mL), 80 °C, 24 h.bConditions: alkene (0.2 mmol), PdCl2(5 mol%), Xantphos (6 mol%), Ph2tBuSiCl (0.3 mmol), AcOH (0.3 mmol), CO (40 atm), PhCl (1.5 mL), 100 °C, 24 h.c100 °C. Yields refer to isolated yields of the derivatized methyl carboxylates (see SI). The ratios of regioisomers within parentheses were determined by GC-MS analysis of their derivatized methyl carboxylates of crude acid chlorides. Fig. 4: Synthetic application of hydrochlorocarbonylation. Conditions for a , b , left column: alkene (0.2 mmol), Pd(P t Bu 3 ) 2 (5 mol%), Ph 2 t BuSiCl (0.3 mmol), AcOH (0.3 mmol), CO (30 atm), DCE (1.5 mL), 80 °C, 24 h. Conditions for a , b , right column and c : alkene (0.2 mmol), PdCl 2 (5 mol%), Xantphos (6 mol%), Ph 2 t BuSiCl (0.3 mmol), AcOH (0.3 mmol), CO (40 atm), PhCl (1.5 mL), 100 °C, 24 h. After completed the hydrochlorocarbonylation, the crude acid chloride was involved in follow-up acylation with the corresponding nucleophiles in one-pot. Isolated yields. Full size image One-pot hydrochlorocarbonylation and amidation with aliphatic amines have subsequently been studied (Fig. 4b ). Aliphatic amines and 2-aminopyridine that inhibit the generation of active metal-hydride catalyst in hydroaminocarbonylation reactions, could be easily transformed into amides 5g–5k and 6g–6k in good to high yields in one-pot hydrochlorocarbonylation-amidation reactions. Additionally, as illustrated in 5l–5n and 6l–6n , one-pot hydrochlorocarbonylation-thioesterification, one-pot hydrochlorocarbonylation-C-C bond coupling reaction, and one-pot hydrochlorocarbonylation-Friedel-Crafts acylation were proceeded smoothly, thus demonstrating the usefulness of this Pd-catalyzed hydrochlorocarbonylation of alkenes. In order to further demonstrate the utility of the hydrochlorocarbonylation, late-stage functionalization of complex bioactive molecules has been examined (Fig. 4c ). Delightfully, the hydrochlorocarbonylation showed high efficiency in these cases, following by one-pot esterification/amidation, the ester/amide 7a–7c that linked two bioactive molecules were obtained in 63–78% yield. Mechanistic studies To gain mechanistic insight into the reaction, control experiments were performed. When the reaction was operated in a two-chamber system with the ex situ generation of HCl from tert-butylchlorodiphenylsilane and AcOH, a 56% yield of acid chloride 2a was obtained (Fig. 5a (a) ). This result suggested that tert-butylchlorodiphenylsilane combined with AcOH play a role as mild HCl-releasing reagents. To check if the reaction started from a palladium-hydride insertion pathway or a hydrochlorination pathway, (1-chloroethyl)benzene 8 was used as the substrate in the reaction (Fig. 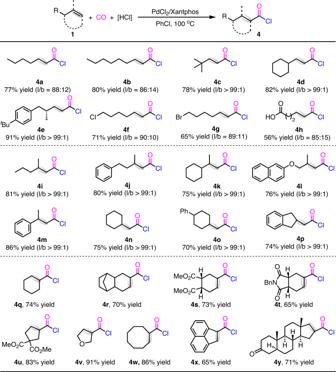Fig. 3: Pd-catalyzed hydrochlorocarbonylation of various alkenes. Conditions: alkene (0.2 mmol), PdCl2(5 mol%), Xantphos (6 mol%), Ph2tBuSiCl (0.3 mmol), AcOH (0.3 mmol), CO (40 atm), PhCl (1.5 mL), 100 °C, 24 h. Isolated yields of the derivatized products (see SI). The ratio of isomers within parentheses was determined by GC-MS analysis of the derivatized products of the acid chlorides. 5a (b) ). The result of no reaction in this case indicated that the hydrochlorination of alkene was excluded from our hydrochlorocarbonylation. Fig. 5: Mechanistic studies. a Two chamber experiments. b Tentative mechanisms of the reaction. c Control experiment. Full size image As a result, tentative mechanisms that proceeded through palladium hydride pathway were proposed in Fig. 5b . Initially, coordination and insertion of alkene 1 into palladium hydride A affords the alkyl-Pd-Cl intermediate B . The alkyl-Pd-Cl B undergoes CO coordination and insertion to generate the acyl-Pd-Cl intermediate C . Reductive elimination of acyl-Pd-Cl species C produces the desired acid chloride and palladium catalyst Pd(0)L. Finally, oxidative addition of Pd(0)L into HCl forms the palladium hydride catalyst A (path a). Alternatively, the catalytic cycle might be directly completed to form the acid chloride and palladium hydride A through chlorolysis of acyl-Pd-Cl intermediate C by HCl (path b). In both catalytic cycles, the regiocontrol were dependent on the ligand and solvent. To identify above two catalytic cycles, further studies have been conducted. First, the acyl-palladium complex 9 , a stable and yellow precipitate [19] , was prepared by the reaction of 3a and stoichiometric Pd(P t Bu 3 ) 2 in n -hexane (Fig. 5c (a) ). Stirring the acyl-palladium 9 in DCE solvent at room temperature in 1 h, 23% yield of styrene 10 was formed (Fig. 5c (b) ). Similar result was observed under 2.0 equiv of HCl. However, when the reaction was operated under balloon pressure of CO, the acid chloride 3a was obtained in 29% yield. And the yield of acid chloride 3a was enhanced to 66% under high pressure of CO [51] . These observations suggested that: (1) the pathway of chlorolysis of acyl-Pd-Cl intermediate C to form acid chloride (Fig. 5b , path b) is less likely; (2) CO prompted reductive elimination of acyl-palladium species 9 to afford acid chloride is reasonable (Fig. 5b , path a); and (3) both the step of insertion of palladium hydride A into alkenes and insertion of CO into alkyl-Pd intermediate B are irreversible under CO [42] , [52] , [53] . In summary, we have developed a novel and effective palladium-catalyzed hydrochlorocarbonylation of alkenes for the synthesis of alkyl acid chlorides. Depended on the ligands and solvents, both branched and linear alkyl acid chlorides were formed selectively in good to high yields. The reaction employs tert-butylchlorodiphenylsilane and AcOH as mild HCl source and shows good functional group compatibility. Cooperating with follow-up acylation reactions, this Pd-catalyzed hydrochlorocarbonylation offers a complementary platform for the synthesis of diverse carbonyl compounds from readily available alkenes. Mechanistic investigations revealed that the reaction proceeded through a palladium hydride mechanism, and CO prompted reductive elimination of the acyl-Pd-Cl intermediate. Synthesis of compound 2 In a glove box, to a dry and stirred glass vessel, alkene 1 (0.2 mmol, 1.0 equiv), Pd(P t Bu 3 ) 2 (0.01 mmol, 5 mol%), and DCE (1.5 mL) were added. To the above mixture, Ph 2 t BuSiCl (0.3 mmol, 1.5 equiv) and AcOH (0.3 mmol, 1.5 equiv) were added. The glass vessel was then put into an autoclave. 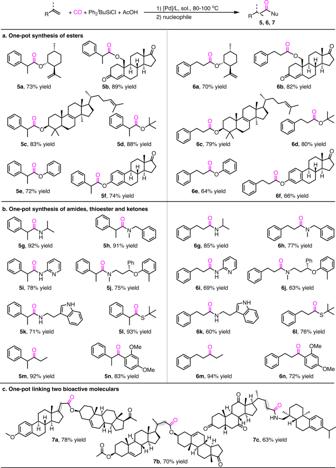Fig. 4: Synthetic application of hydrochlorocarbonylation. Conditions fora,b, left column: alkene (0.2 mmol), Pd(PtBu3)2(5 mol%), Ph2tBuSiCl (0.3 mmol), AcOH (0.3 mmol), CO (30 atm), DCE (1.5 mL), 80 °C, 24 h. Conditions fora,b, right column andc: alkene (0.2 mmol), PdCl2(5 mol%), Xantphos (6 mol%), Ph2tBuSiCl (0.3 mmol), AcOH (0.3 mmol), CO (40 atm), PhCl (1.5 mL), 100 °C, 24 h. After completed the hydrochlorocarbonylation, the crude acid chloride was involved in follow-up acylation with the corresponding nucleophiles in one-pot. Isolated yields. 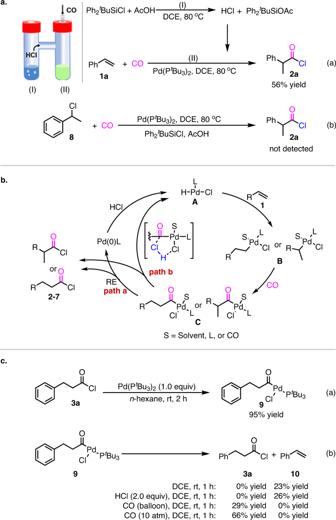Fig. 5: Mechanistic studies. aTwo chamber experiments.bTentative mechanisms of the reaction.cControl experiment. The autoclave was evacuated and backfilled with CO for three times in a well-ventilated fume hood and then pressurized to 30 atm of CO. The reaction mixture in autoclave was stirred at 80 °C for 24 h. After the reaction completed, the autoclave was cooled down to room temperature. Then, the CO in autoclave was carefully released in a well-ventilated fume hood. Take out the glass vessel, and MeOH (1.0 mL) was added. The mixture in glass vessel was stirred for 30 mins at room temperature. The residue was purified by column chromatography on silica gel to afford the corresponding methyl carboxylate by flash column chromatography on silica gel. Synthesis of compound 3 In a glove box, to a dry and stirred glass vessel, alkene 1 (0.2 mmol, 1.0 equiv), PdCl 2 (0.01 mmol, 5 mol%), Xantphos (0.012 mmol, 6 mol%) and PhCl (1.5 mL) were added. To the above mixture, Ph 2 t BuSiCl (0.3 mmol, 1.5 equiv) and AcOH (0.3 mmol, 1.5 equiv) were added. The glass vessel was then put into an autoclave. The autoclave was evacuated and backfilled with CO for three times in a well-ventilated fume hood and then pressurized to 40 atm of CO. The reaction mixture in autoclave was stirred at 100 °C for 24 h. After the reaction completed, the autoclave was cooled down to room temperature. Then, the CO in autoclave was carefully released in a well-ventilated fume hood. Take out the glass vessel, and MeOH (1.0 mL) was added. The mixture in glass vessel was stirred for 30 mins at room temperature. The residue was purified by column chromatography on silica gel to afford the corresponding methyl carboxylate by flash column chromatography on silica gel.